New evidence on the colour and nature of the isolatedArchaeopteryxfeather Archaeopteryx has been regarded as an icon of evolution ever since its discovery from the Late Jurassic limestone deposits of Solnhofen, Germany in 1861. Here we report the first evidence of colour from Archaeopteryx based on fossilized colour-imparting melanosomes discovered in this isolated feather specimen. Using a phylogenetically diverse database of extant bird feathers, statistical analysis of melanosome morphology predicts that the original colour of this Archaeopteryx feather was black, with 95% probability. Furthermore, reexamination of the feather's morphology leads us to interpret it as an upper major primary covert, contrary to previous interpretations. Additional findings reveal that the specimen is preserved as an organosulphur residue, and that barbule microstructure identical to that of modern bird feathers had evolved as early as the Jurassic. As in extant birds, the extensive melanization would have provided structural advantages to the Archaeopteryx wing feather during this early evolutionary stage of dinosaur flight. In 1861, Archaeopteryx lithographica was unearthed from the 150-million-year-old Solnhofen Lagerstätte [1] . The mosaic of reptilian traits (for example, teeth, long vertebral tail and manual unguals) and avian plumage in these fossils ( Fig. 1a,b ) has since inspired a rich scientific literature on Archaeopteryx and the origin of birds [1] , [3] , yet the animal's colour, a diverse and multifunctional trait in modern birds [4] , [5] , [6] , has remained only speculative. Additionally, unresolved questions have persisted regarding the anatomical identity and composition of the isolated feather specimen, which was the first described Archaeopteryx fossil [7] , [8] , [9] and the only one preserved as a dark trace ( Fig. 1a ) [1] , [10] , [11] . 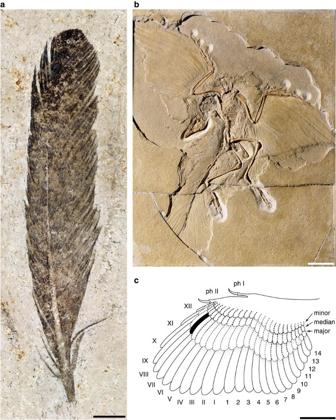Figure 1: Specimens and reconstructed wing ofArchaeopteryx. (a) Optical photograph of the isolated fossil feather (MB.Av.100). Scale bar: 5 mm. (b) Berlin skeletal specimen (HMN 1880), showing the ventral surface of the wings1,2. Scale bar: 5 cm. (c) Dorsal surface of left wing showing approximate location of isolated feather (in black), interpreted as a distal member of the major tract of upper primary coverts. Wing redrawn after Wellnhofer1, based on the Berlin skeleton and showing phalanges (ph I,II), primaries (I–XII), secondaries (1–14) and hypothetical reconstructions of major, median and minor tracts of upper coverts (dashed lines)1. Scale bar: 5 cm. Figure 1: Specimens and reconstructed wing of Archaeopteryx . ( a ) Optical photograph of the isolated fossil feather (MB.Av.100). Scale bar: 5 mm. ( b ) Berlin skeletal specimen (HMN 1880), showing the ventral surface of the wings [1] , [2] . Scale bar: 5 cm. ( c ) Dorsal surface of left wing showing approximate location of isolated feather (in black), interpreted as a distal member of the major tract of upper primary coverts. Wing redrawn after Wellnhofer [1] , based on the Berlin skeleton and showing phalanges (ph I,II), primaries (I–XII), secondaries (1–14) and hypothetical reconstructions of major, median and minor tracts of upper coverts (dashed lines) [1] . Scale bar: 5 cm. Full size image Similar fossilized feather traces have been found to preserve colour-imparting organelles called melanosomes [12] , [13] , [14] , [15] , [16] , which consist of melanins, the most widespread and abundant pigments in animals and found in the feathers of all birds (excluding albinos) [4] . Melanins primarily fall into two categories, eumelanins and phaeomelanins [4] , and the morphological properties of the associated melanosomes have been used to reconstruct various plumage colours of extinct dinosaurs [12] , [13] , [14] , [15] , [16] . Elucidating the phylogenetic and anatomical distributions of feather colouration can further our understanding of dinosaur evolution, palaeobiology and aesthetics. Here we provide the first evidence of colour from Archaeopteryx , along with new information regarding the identity, preservation and microstructure of the isolated feather. Identity The specimen is considered to be a wing feather with aerodynamic function, based on its vane asymmetry [9] , [10] , [17] , [18] , lateral curvature [17] and obtusely angled distal tip [10] . In particular, the feather has previously been identified as a distal secondary [1] , [10] or distal primary [19] . However, compared with the secondary and primary feathers of the skeletal specimens, the isolated feather is much wider relative to its length [10] . Furthermore, either interpretation would require that this small, moulted [1] , [2] , [10] feather originated from an individual much smaller than the other known Archaeopteryx specimens [2] , [10] , [20] , which all represent immature individuals [21] , [22] . However, previous interpretations did not consider the relatively long calamus, which was originally visible on the specimen as a faint trace [9] but has since worn away [20] . While the mode of feather attachment in Archaeopteryx is unknown [20] , comparison of the relative calamus length (22% of total feather length, 1.5 cm/6.9 cm) [9] to that of modern bird feathers [23] suggests that the specimen may represent a distal member of the upper major primary coverts ( Fig. 1c ). With respect to other wing coverts, this particular interpretation of the feather is further supported by its angled distal tip [10] as well as the asymmetric and almost entirely closed pennaceous nature of its vanes [23] . Our interpretation is also more consistent with the relative width and small size of the feather, and would imply that the specimen was from the wing of an individual within the size range of the skeletal specimens of Archaeopteryx (presuming that the feather is conspecific [1] ). Preservation We interpret the feather's dark trace to be a melanic organosulphur residue, based on the following. First, we detected no manganese among nine point analyses throughout the feather, indicating that preservation was not due to precipitation of the inorganic mineral, manganese dioxide (MnO 2 ), as has been suggested by some workers [1] , [2] , [10] , [24] . Second, a potential organocopper biomarker for melanin was previously detected in this specimen; this biomarker has also been correlated with the presence of melanosomes in three fossil bird taxa [25] . We hypothesize that melanosome structures fossilize simply by virtue of being solid aggregations of melanins [26] , [27] , [28] , which themselves have high preservation potential [29] as large, insoluble polymers resistant to degradation [4] . Third, the dark trace is associated with sulphur ( Fig. 2 ), which may have derived from the sulphur-rich feather keratin [23] , [25] and crosslinked with the melanin [4] ; this is consistent with the sulphurization mechanism responsible for high-fidelity organic preservation in the fossil record [30] . Indeed, the dark trace preserves very fine details of the feather barbs and barbules ( Fig. 2b ). 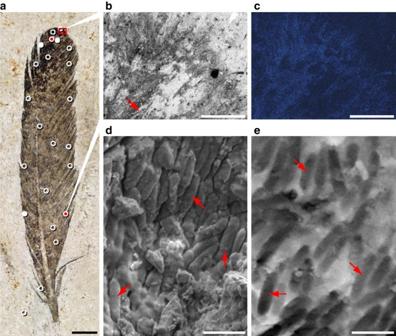Figure 2: Organosulphur residue and melanosomes in theArchaeopteryxfeather. (a) Optical photograph indicating sample locations (circles; not to scale) examined via SEM. Red-filled circles (n=2) represent locations where data were collected for statistical analysis (Supplementary Fig. S1). White-filled circles (n=4) represent locations where melanosomes were observed but not measured due to poor preservation; unfilled circles (n=17) represent locations where no melanosomes were observed. Scale bar: 5 mm. (b) Detail of boxed area (a), backscattered electron image showing barb and barbule (arrow) microstructure preserved as melanic organosulphur residue. Scale bar: 500 μm. (c) Detail of boxed area (a), spectral X-ray map for sulphur Kα; blue and black correspond to higher and lower intensities (concentrations), respectively. Scale bar: 500 μm. (d,e) SEM images taken from location of proximal red-filled circle (a), showing melanosomes (arrows) preserved three-dimensionally and as moulded imprints, respectively. Scale bars: 1 μm. Figure 2: Organosulphur residue and melanosomes in the Archaeopteryx feather. ( a ) Optical photograph indicating sample locations (circles; not to scale) examined via SEM. Red-filled circles ( n =2) represent locations where data were collected for statistical analysis ( Supplementary Fig. S1 ). White-filled circles ( n =4) represent locations where melanosomes were observed but not measured due to poor preservation; unfilled circles ( n =17) represent locations where no melanosomes were observed. Scale bar: 5 mm. ( b ) Detail of boxed area ( a ), backscattered electron image showing barb and barbule (arrow) microstructure preserved as melanic organosulphur residue. Scale bar: 500 μm. ( c ) Detail of boxed area ( a ), spectral X-ray map for sulphur Kα; blue and black correspond to higher and lower intensities (concentrations), respectively. Scale bar: 500 μm. ( d , e ) SEM images taken from location of proximal red-filled circle ( a ), showing melanosomes (arrows) preserved three-dimensionally and as moulded imprints, respectively. Scale bars: 1 μm. Full size image Microstructure Barbules are also preserved as topographic impressions within the limestone matrix, and are indistinguishable from those of modern pennaceous feathers with respect to morphology [23] and barbule angles [31] ( Fig. 3 ). These impressions include a parallel array of distal barbules ( Fig. 3b ) that contain moulded imprints of melanosomes. Other melanosome imprints are aligned along the longitudinal axis of a proximal barbule ( Fig. 3c,d ), an arrangement previously reported in the barbules of extant and more recent fossil bird feathers [14] , [15] . 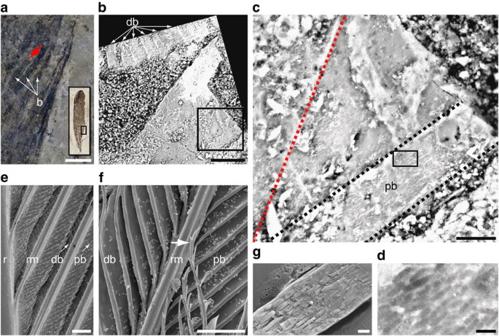Figure 3: Barbule microstructure inArchaeopteryxand extant bird feathers. (a) Optical photograph of boxed area within theArchaeopteryxfeather (inset). Scale bar: 1 mm. (b) SEM image from (a, red arrow) showing topographic impressions of a parallel array of distal barbules and a proximal barbule (boxed area). Scale bar: 50 μm. (c) Detail of boxed area (b). Dashed black lines indicate ridges of proximal barbule; dashed red line indicates possible ridge of corresponding barb ramus. Scale bar: 10 μm. (d) Detail of boxed area (c), showing rod-shaped melanosome imprints aligned along longitudinal axis of barbule. Scale bar: 1 μm. (e,f) SEM images of barbs from a primary covert (ventral and dorsal surfaces, respectively) of American Woodcock (Scolopax minor). Arrow (f) indicates barbicel of overlapping distal barbule from adjacent barb; neighbouring distal barbules to the right have been removed to expose underlying proximal barbules. Scale bars: 100 μm (e) and 50 μm (f). (g) SEM image of longitudinal cross-section from barbule of White-breasted Nuthatch (Sitta carolinensis), showing alignment of melanosomes along longitudinal axis of barbule. Scale bar: 1 μm. Abbreviations: b, barb; db, distal barbule; pb, proximal barbule; r, rachis; rm, ramus. Figure 3: Barbule microstructure in Archaeopteryx and extant bird feathers. ( a ) Optical photograph of boxed area within the Archaeopteryx feather (inset). Scale bar: 1 mm. ( b ) SEM image from ( a , red arrow) showing topographic impressions of a parallel array of distal barbules and a proximal barbule (boxed area). Scale bar: 50 μm. ( c ) Detail of boxed area ( b ). Dashed black lines indicate ridges of proximal barbule; dashed red line indicates possible ridge of corresponding barb ramus. Scale bar: 10 μm. ( d ) Detail of boxed area ( c ), showing rod-shaped melanosome imprints aligned along longitudinal axis of barbule. Scale bar: 1 μm. ( e , f ) SEM images of barbs from a primary covert (ventral and dorsal surfaces, respectively) of American Woodcock ( Scolopax minor ). Arrow ( f ) indicates barbicel of overlapping distal barbule from adjacent barb; neighbouring distal barbules to the right have been removed to expose underlying proximal barbules. Scale bars: 100 μm ( e ) and 50 μm ( f ). ( g ) SEM image of longitudinal cross-section from barbule of White-breasted Nuthatch ( Sitta carolinensis ), showing alignment of melanosomes along longitudinal axis of barbule. Scale bar: 1 μm. Abbreviations: b, barb; db, distal barbule; pb, proximal barbule; r, rachis; rm, ramus. Full size image Colour Only rod-shaped eumelanosomes were observed in the Archaeopteryx feather (including melanosomes that were not measured), and are preserved both as imprints (~0.53–1.7 μm long, 180–360 nm wide, n =86) and as three-dimensional (3D) structures (~0.55–1.2 μm long, 140–280 nm wide, n =22) ( Fig. 2d,e ; Supplementary Table S1 ). Long and short axes are significantly greater in imprints than in 3D melanosomes (both P -values <0.001), as previously reported [12] , and the aspect ratio of imprints is significantly smaller ( P -value=0.034). Based on statistical analysis of five properties of melanosome morphology, we predict the original colour of the Archaeopteryx feather to be black, with 95% probability ( Fig. 4 ). Separate analyses of imprints and 3D melanosomes also predict black colouration, with 91 and 75% probability, respectively. 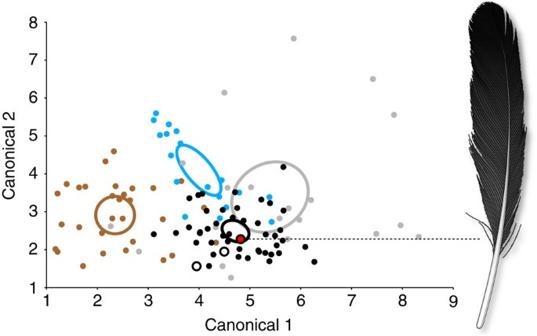Figure 4: Statistical analysis for reconstructingArchaeopteryxfeather colour. Quadratic discriminant analysis of brown, black, grey and penguin type12from extant birds (solid points,n=115;Supplementary Table S2) andArchaeopteryx(red-filled black circle; two unfilled black circles denote each melanosome preservation type analysed separately). Data points and 95% confidence bounds (ellipses) are shown in the colour of their respective classes; penguin type is shown in blue. Morphology of reconstructed feather is based on von Meyer (Plate VIII,Fig. 3)9; note original calamus length relative to that inFigure 1a. Figure 4: Statistical analysis for reconstructing Archaeopteryx feather colour. Quadratic discriminant analysis of brown, black, grey and penguin type [12] from extant birds (solid points, n =115; Supplementary Table S2 ) and Archaeopteryx (red-filled black circle; two unfilled black circles denote each melanosome preservation type analysed separately). Data points and 95% confidence bounds (ellipses) are shown in the colour of their respective classes; penguin type is shown in blue. Morphology of reconstructed feather is based on von Meyer (Plate VIII, Fig. 3 ) [9] ; note original calamus length relative to that in Figure 1a . Full size image Herein we have provided the first evidence of colour from Archaeopteryx , and have demonstrated that the isolated fossil feather is most likely an upper major primary covert, exhibits modern barbule microstructure, and is preserved as an organosulphur residue. It is improbable that either of the other major classes of feather pigments, carotenoids and porphyrins, were also present in the Archaeopteryx feather, as they are relatively uncommon [4] and generally do not occur in flight feathers, presumably for structural reasons [23] , [32] . Additionally, even if there were codeposition of another pigment, the black melanin would likely mask its presence [4] . Indeed, the melanic residue is ubiquitous throughout the feather vanes, and no banding patterns [15] are visible. We do not consider minor variation in local residue abundance to be indicative of pigmentation patterns [24] , as light and dark areas often correspond to dark and light areas in the specimen's counterpart (BSP 1869 VIII 1), respectively (see Fig. 5.7 in Wellnhofer [1] ); missing barbs are often preserved on the counterpart as well [24] . However, the residue does appear darkest at the distal tip of both this specimen ( Fig. 1a ) and its counterpart [9] , which may reflect a greater degree of melanization in this region. The black pigmentation observed in areas of the feather not generally visible during the animal's life, such as the proximal region obscured by overlapping covert feathers ( Fig. 1c ) and proximal barbules obscured by overlapping distal barbules ( Fig. 3c,e,f ), suggests at least a partially non-visual role for this melanization [23] . Although black pigmentation in the wing may have had a role in the crypsis, communication and/or thermoregulation [4] of Archaeopteryx , such inferences cannot be made with any certainty. Similarly, in modern birds, melanins confer protection against feather-degrading bacteria that flourish in humid habitats [4] , [33] , [34] , but it is uncertain whether the dry climate of the Jurassic Solnhofen [1] , [35] would have provided sufficient evolutionary pressure to select for such an adaptation. Nonetheless, melanins are large polymers that strongly crosslink with proteins [4] , and their presence substantially increases feather keratin hardness (by ~39% (ref. 36 )), thickness and resistance to fracture from abrasion and cyclical loading during flight [4] , [5] , [6] , [23] , [36] , [37] . This accounts for the fact that wing feathers (and especially their distal tips, where aerodynamic forces are high) display the greatest tendency towards melanization [4] , [5] , [6] , [38] . The melanization observed throughout the Archaeopteryx wing feather would have provided similar structural advantages during this early evolutionary stage of dinosaur flight. Fossil specimen The isolated Archaeopteryx feather is specimen MB.Av.100, housed at the Humboldt Museum für Naturkunde in Berlin, Germany. The main slab (not analysed in this study) is BSP 1869 VIII 1, housed at the Bayerische Staatssammlung für Paläontologie und Geologie in Munich, Germany. MB.Av.100 has always been the darker of the two feather traces, although it is considered to be the counter slab owing to its original position in the rock (Schwarz-Wings, personal communication). The isolated feather was the original holotype of the nominal species, Archaeopteryx lithographica von Meyer [1] , [8] ; the London specimen (BMNH 37001, housed at the Natural History Museum in London, England) has recently been designated as the neotype [39] . Scanning electron microscopy The feather specimen was examined uncoated using a Zeiss Supra 55VP field emission gun scanning electron microscope (FE-SEM) equipped with an Oxford INCA Energy 300 SEM-energy dispersive X-ray spectroscopy system, at the Carl Zeiss Nanotechnology Center in Oberkochen, Germany. Melanosome imprints were imaged using an angle-selected backscattered detector at 20.00 kV and variable vacuum pressure ( Supplementary Fig. S1a–e ). Melanosomes preserved three-dimensionally were imaged using a secondary electron detector at 1.80 kV and high vacuum pressure ( Supplementary Fig. S1g–l ); one additional image used in the analysis was acquired using a Zeiss Ultra Plus FE-SEM at 3.00 kV ( Supplementary Fig. S1f ). ImageJ software ( http://rsbweb.nih.gov/ij/ ) was used to measure long and short axes of melanosomes ( Supplementary Table S1 ). Statistical analysis Measurements of imprints and 3D melanosomes from the Archaeopteryx feather ( Supplementary Table S1 ) were compared with a two-tailed Student's t -test for long and short axes (homoscedastic) and a two-tailed Welch's t -test for aspect ratios (heteroscedastic) using Microsoft Excel. Melanosome data from 115 extant bird feathers ( Supplementary Table S2 ) were collected and analysed using quadratic discriminant analysis as previously described [12] , [13] . These samples represent a phylogenetically diverse range of 87 taxa from 27 orders, and included 56 additions that approximately doubled the sample size of the previous database. Extant bird samples were predicted to four classes (brown, black, grey and penguin type) based on five properties of melanosome morphology and with 80% cross-validation accuracy. Significant ( α =0.10) discriminating variables of melanosome morphology included long axis ( P -value <0.001), short axis ( P -value <0.001), short axis variation ( P -value <0.001), aspect ratio skew ( P -value=0.008) and long axis skew ( P -value=0.060). The discriminant function was highly significant (Pillai's trace, F 15,324 =11.24, P -value <0.001). Canonical axis 1 explained 71.32% of the variation and was most strongly associated with long axis; canonical axis 2 explained 17.23% of the variation and was most strongly associated with short axis. How to cite this article: Carney, R. M. et al . New evidence on the colour and nature of the isolated Archaeopteryx feather. Nat. Commun. 3:637 doi: 10.1038/ncomms1642 (2012).